Subduction of the oceanic Hikurangi Plateau and its impact on the Kermadec arc Large igneous province subduction is a rare process on Earth. A modern example is the subduction of the oceanic Hikurangi Plateau beneath the southern Kermadec arc, offshore New Zealand. This segment of the arc has the largest total lava volume erupted and the highest volcano density of the entire Kermadec arc. Here we show that Kermadec arc lavas south of ~32°S have elevated Pb and Sr and low Nd isotope ratios, which argues, together with increasing seafloor depth, forearc retreat and crustal thinning, for initial Hikurangi Plateau—Kermadec arc collision ~250 km north of its present position. The combined data set indicates that a much larger portion of the Hikurangi Plateau (the missing Ontong Java Nui piece) than previously believed has already been subducted. Oblique plate convergence caused southward migration of the thickened and buoyant oceanic plateau crust, creating a buoyant ‘Hikurangi’ mélange beneath the Moho that interacts with ascending arc melts. The formation of large igneous provinces (LIPs) represents one of the most extreme volcanic events on Earth, characterized through eruption of vast amounts of lava in a geologically short period [1] . Oceanic LIPs either accrete and obduct, adding to the continental landmass [2] , [3] , [4] or in rare cases recycle back into the Earth’s mantle via subduction. Known examples of oceanic plateau subduction include the Cretaceous Caribbean Plateau, accreting at and subducting/underthrusting beneath the Greater Antilles on the Caribbean Plate and the south-eastern part of the Ontong Java Plateau presently subducting beneath the Solomon Islands at the north Solomon–Kilinailau trench. Both examples involve complex tectonic processes, such as impact-related accretion of oceanic plateau crust and the change of subduction polarity [5] , [6] , [7] , [8] . However, subduction of one tectonic plate beneath another has driven geochemical cycling and the formation of the Earth’s crust since ~3,500 Myr [9] . It has been known for decades that volcanic arcs are the result of that subduction process, as the descending plate dehydrates, causing partial melting in the overlying mantle. Consequently, arc lavas carry geochemical signals from the subducting plate, which includes the sediment cover, altered oceanic crust and serpentinized mantle [10] , [11] , [12] . In addition, signals of subducting intraplate seamounts (or LIPs) with geochemical compositions different to the subarc mantle can be traced in arc lavas [13] , [14] . Tracing the subduction cycle of such geological features provides an improved understanding of mantle-flow pattern and may explain the variability in eruptive behaviour and style of hydrothermal activity on the overriding plate [15] . A globally unique example of single polarity oceanic plateau subduction is the Hikurangi Plateau presently subducting beneath the southern Kermadec arc and the North Island of New Zealand ( Fig. 1 ) [16] , [17] , [18] , [19] . Subduction of 15–23-km thick, altered and buoyant Hikurangi Plateau crust, that is host to large seamounts [19] , [20] , must not only have a strong effect on tectonic erosion and the local plate stress regime, but also on volatile element budgets in the overlying mantle. This in turn suggests significant implications for the petrogenesis and eruptive behaviour of arc volcanoes, fluid-flow in their associated hydrothermal systems, and element transfer to the oceans. The Hikurangi Plateau is believed to have formed as part of Ontong Java Nui during the ‘greater Ontong Java event’ ~120 Myr ago, one of the world’s most extreme volcanic events, covering ~1% of the Earth’s surface [18] , [21] , [22] . As noted by Chandler et al. [22] , a large part of the Hikurangi Plateau connecting its western and northern margin with the Ontong Java and Manihiki plateaus either does not exist or has already been subducted. 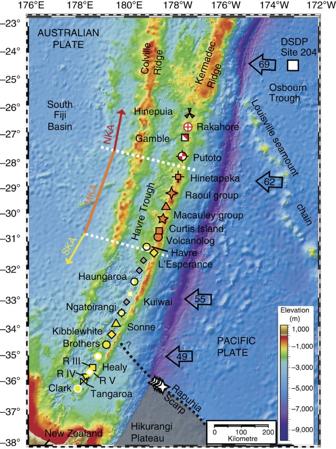Figure 1: Bathymetric map of the Kermadec arc—Havre Trough backarc system. Symbols mark the Kermadec arc volcanic centre locations discussed in this paper, with coloured symbols used for the different volcanic centres from which isotopic data are available; the grey symbols are for volcanoes for which no isotope data are available. White stars mark the location of additional Hikurangi Plateau samples used in this study. The numbers in the arrows are subduction velocities, as in ref.23. For the purpose of this study we separate the Kermadec arc into three segments on the basis of the location of the volcanic front behind or on the Kermadec Ridge: (1) the northern Kermadec arc (NKA) between ~25° and 28.5°S, (2) the mid Kermadec arc (MKA) between ~29 and ~32°S and (3) the southern Kermadec arc (SKA) between 32° and 37°S. DSDP, Deep Sea Drilling Programme. Figure 1: Bathymetric map of the Kermadec arc—Havre Trough backarc system. Symbols mark the Kermadec arc volcanic centre locations discussed in this paper, with coloured symbols used for the different volcanic centres from which isotopic data are available; the grey symbols are for volcanoes for which no isotope data are available. White stars mark the location of additional Hikurangi Plateau samples used in this study. The numbers in the arrows are subduction velocities, as in ref. 23 . For the purpose of this study we separate the Kermadec arc into three segments on the basis of the location of the volcanic front behind or on the Kermadec Ridge: (1) the northern Kermadec arc (NKA) between ~25° and 28.5°S, (2) the mid Kermadec arc (MKA) between ~29 and ~32°S and (3) the southern Kermadec arc (SKA) between 32° and 37°S. DSDP, Deep Sea Drilling Programme. Full size image In this study we present new Sr-, Nd-, and Pb-isotope data from Kermadec arc and Hikurangi Plateau lavas ( Fig. 1 ) which, when combined with published isotope and satellite gravity data and bathymetry, show large-scale geochemical and geophysical variations along the length of the Kermadec arc, enabling us to better understand the processes related to LIP subduction and thus identifying the ‘missing’ piece of Ontong Java Nui. Geological background The ~1,300-km long, intra-oceanic, mostly submarine Kermadec arc system results from Pacific–Australian Plate convergence and forms the southern part of the Tonga–Kermadec arc system that extends ~2,500 km north of New Zealand. The Kermadec arc is one of the worlds most volcanically and hydrothermally active arc systems, with ~75% of the 33 major volcanoes being hydrothermally active [15] . Subduction velocities decrease from the fastest convergence rates on Earth of ~24 cm per year at the northern end of the Tonga arc system [23] , to ~5 cm per year along the southern Kermadec arc. The sediment veneer on the incoming Pacific Plate, changes in thickness and composition from ~200 m of pelagic sediments near ~25°S (that is, DSDP Site 204; for example, ref. 24 ; Fig. 1 ) to ≥500 m of predominantly terrigeneous sediments near ~36°S (ref. 25 ). North of ~28.5°S, the Kermadec arc front volcanoes are located in the Havre Trough backarc immediately west of the relatively old and inactive Kermadec Ridge before they merge with the Kermadec Ridge between ~29°S and ~32°S. At ~32°S, the arc front shows a sudden ~15 km offset into the Havre Trough accompanied by ~500 m average seafloor deepening [15] , [26] . South of 32°S, the majority of the volcanic front volcanoes are located behind the Kermadec Ridge and the forearc narrows by ~75 km from a gently trenchward dipping and ~200-km wide to ~125-km wide [27] . These authors also inferred a westward trench retreat of ≤50 km, and that the forearc inner trench margin south of 32°S subsided by ≤4 km, summing up to a loss in volume of ~400 km 3 compared with the north. South of ~35°S, subduction of the Cretaceous Hikurangi Plateau beneath the southern Kermadec arc is accompanied by an average shoaling of ~500 m of the Kermadec forearc, arc front and Havre Trough backarc [15] , [28] , [29] . The plateau hosts ≤2,900 m high ridge-like seamounts and guyots with basal diameters ≤25 km. Two-dimensional gravity modelling and estimates from active seismic source refraction studies suggests a Hikurangi Plateau crustal thickness of 15–23 km compared with a 4–6 km thick Pacific oceanic crust to the north [18] , [30] , [31] . Both these techniques assume that the mantle is marked by either Vp seismic velocities >8 km s −1 or densities >3.0 × 10 3 kg m −3 . Reyners et al. [20] however identified a seismically active 35-km thick layer beneath the upper surface of the subducting Hikurangi Plateau. The presence of >8.5 km s −1 velocities at the base of the seismically active zone led Reyners et al. [20] to propose an eclogite layer to the plateau ‘crust’, doubling the thickness modelled by Davy et al. [18] and Scherwarth et al. [30] Geochemistry Lava compositions from the Kermadec arc volcanoes range from basalt to rhyolite within the low-K tholeiitic to medium-K calcalkaline series (e.g. refs 29 , 32 ), following the rock classification by Le Maitre [33] and show typical subduction zone enrichments of elements mobile in aqueous fluids (for example, Rb, Ba, U, Pb, Sr) and depletions in Nb when compared with mid-ocean ridge basalts (MORB [34] ). Of all the Kermadec arc front lavas, those from the northern Kermadec arc volcanoes between 26 and 28°S show the least radiogenic values for Pb and Sr (for example, 206 Pb/ 204 Pb Avg =18.67; 87 Sr/ 86 Sr Avg =0.7034; see Table 1 for Sr-, Nd- and Pb-isotope data) and fall between Pacific MORB and sediments drilled at DSDP Site 204 (refs 24 , 35 ; Fig. 2a,c ). The northern Kermadec arc lavas are also characterized by Pacific MORB-like (most radiogenic) Nd isotopic compositions ( 143 Nd/ 144 Nd Avg =0.5131; Fig. 2b ). A noticeable increase in average Pb and Sr isotopic composition to 206 Pb/ 204 Pb Avg =18.69 and 87 Sr/ 86 Sr Avg =0.7036, and a decrease in 143 Nd/ 144 Nd Avg to 0.51304, is shown by lavas erupted on the Kermadec Ridge. At ~32°S, the arc front lava Pb and Sr isotopic compositions become significantly more radiogenic, yet Nd isotope ratios become less radiogenic (for example, 206 Pb/ 204 Pb Avg =18.84; 87 Sr/ 86 Sr Avg =0.7039; 143 Nd/ 144 Nd Avg =0.512987). South of ~35°S above the presently subducting Hikurangi Plateau, the average Pb-isotope composition is variable but on average slightly less radiogenic than in lavas from adjacent volcanoes further north (for example, 206 Pb/ 204 Pb Avg =18.77), together with slightly higher Sr ( 87 Sr/ 86 Sr Avg =0.7042) and Nd isotope ratios ( 143 Nd/ 144 Nd Avg =0.512988; Fig. 2 ). 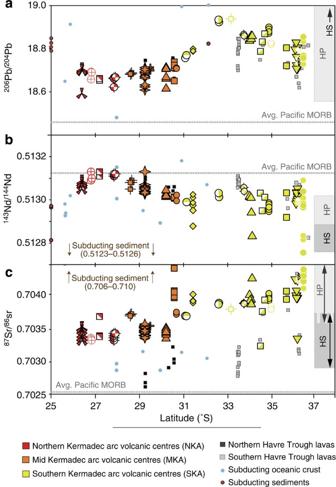Figure 2: Isotopic changes with latitude. Latitude (in °S) versus (a)206Pb/204Pb, (b)143Nd/144Nd, (c)87Sr/86Sr. Yellow symbols mark analyses from southern Kermadec arc (SKA) lavas. Orange symbols represent mid Kermadec arc (MKA) lava analyses and red symbols represent northern Kermadec arc (NKA) lava analyses. HP, Hikurangi Plateau and HS, Hikurangi seamounts (data range as in refs17,19and this study). Average (avg.) Pacific MORB data are from ref.55and references therein. Published Kermadec arc lava data are from refs24,34,35,36,37,56,57,58,59,60. Subducting sediment data are taken from refs24,35,36,56. Altered oceanic crust data are from refs61,62. As discussed in ref.63, the Pb-isotope data set as in ref.24were affected by analytical artefacts leading to lower206Pb/204Pb values outside of the analytical error compared with new analyses on the same samples, and thus were omitted in this compilation. Table 1 Sr–Nd–Pb-isotope data from selected Kermadec arc volcanic centres and the Rapuhia Scarp of the Hikurangi Plateau Full size table Figure 2: Isotopic changes with latitude. Latitude (in °S) versus ( a ) 206 Pb/ 204 Pb, ( b ) 143 Nd/ 144 Nd, ( c ) 87 Sr/ 86 Sr. Yellow symbols mark analyses from southern Kermadec arc (SKA) lavas. Orange symbols represent mid Kermadec arc (MKA) lava analyses and red symbols represent northern Kermadec arc (NKA) lava analyses. HP, Hikurangi Plateau and HS, Hikurangi seamounts (data range as in refs 17 , 19 and this study). Average (avg.) Pacific MORB data are from ref. 55 and references therein. Published Kermadec arc lava data are from refs 24 , 34 , 35 , 36 , 37 , 56 , 57 , 58 , 59 , 60 . Subducting sediment data are taken from refs 24 , 35 , 36 , 56 . Altered oceanic crust data are from refs 61 , 62 . As discussed in ref. 63 , the Pb-isotope data set as in ref. 24 were affected by analytical artefacts leading to lower 206 Pb/ 204 Pb values outside of the analytical error compared with new analyses on the same samples, and thus were omitted in this compilation. Full size image Most lavas from the Kermadec arc volcanic centres show MORB-like less fluid mobile and conservative trace element ratios, but generally high element ratios tracing slab-derived fluids (La/Yb<1; Ba/Th<1,200; refs 24 , 34 ). The Sr and Pb isotopic composition of the northern Kermadec arc lavas have previously been interpreted to show the effects of a MORB-type mantle wedge with the addition of ~1–4% subducted sediment- and altered oceanic crust-derived, fluid-transported isotope signature. Conversely, mantle wedge heterogeneity has been proposed to explain the variations in much less fluid-mobile Nd isotope ratios in northern and southern Kermadec arc lavas [34] , [36] , [37] , [38] . The generally elevated Sr and Pb, and slightly lower Nd isotope ratios in lavas from mid Kermadec arc volcanic centres located on the Kermadec Ridge have been attributed to (1) the interaction of ascending magmas with older Kermadec Ridge crust with higher Pb and Sr, but lower Nd isotopic values compared with the Havre Trough backarc crust [35] , [37] and (2) the input of slab-derived fluids carrying more radiogenic Pb and Sr isotope signatures [34] . Despite their emplacement behind the Kermadec Ridge on Havre Trough backarc crust, the southern Kermadec arc lavas also show elevated Pb and Sr, and low Nd isotopic compositions suggesting an isotopically enriched source beneath these volcanoes. Previously, the increase in Pb and Sr isotope ratios in the southern Kermadec arc lavas were considered to be the result of radiogenic New Zealand-derived terrigenous sediment subduction [37] . However, some lavas between ~32–35°S show higher 206 Pb/ 204 Pb values than local subducting sediment Pb-isotope compositions ( Figs 2a and 3c,d ), requiring an additional high value 206 Pb/ 204 Pb component contributing to the arc lava geochemical compositions. One possible endmember is the nearby subducting Hikurangi Plateau with its large HIMU-type (HIMU=high-time integrated U/Pb ratio) seamounts ( cf. refs 17 , 19 ). Exposure of the ~1-km high Rapuhia Scarp (and deep reaching faults on the Hikurangi Plateau [18] ) and a ≥1.5-km thick layer of sediments/volcaniclastics to seawater alteration for ~120 Myr suggests that parts of the Hikurangi Plateau are more H 2 O-rich than ‘normal’ altered oceanic crust (supported by high and variable contents of large ion lithophile elements [17] , [19] ). 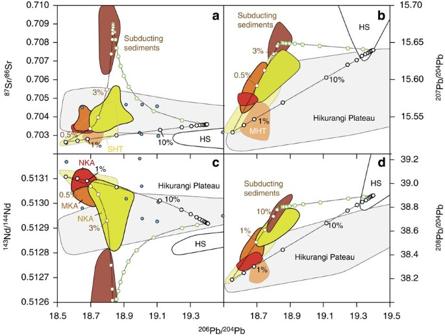Figure 3: Kermadec arc Isotopic variation. 206Pb/204Pb versus a)87Sr/86Sr, b)207Pb/204Pb, c)143Nd/144Nd and d)208Pb/204Pb. Fields shown are for NKA (red), MKA (orange) and SKA (yellow), subducted sediments (red-brown), Hikurangi Plateau (HP; grey) and Hikurangi seamounts (HS; white); MHT, mid Havre Trough; SHT, southern Havre Trough. Dashed lines with hexagons are mixing calculations between; (1) depleted mantle wedge and subducted sediments, (2) depleted mantle wedge and Hikurangi Plateau (consisting of 90% average Hikurangi Plateau basement and 10% average Hikurangi seamounts) and (3) subducted sediments and Hikurangi Plateau. SeeSupplementary Table 1for modelling details. Hikurangi Plateau and seamount data are from refs17,19, and this study. Figure 3: Kermadec arc Isotopic variation. 206 Pb/ 204 Pb versus a) 87 Sr/ 86 Sr, b) 207 Pb /204 Pb, c) 143 Nd/ 144 Nd and d) 208 Pb/ 204 Pb. Fields shown are for NKA (red), MKA (orange) and SKA (yellow), subducted sediments (red-brown), Hikurangi Plateau (HP; grey) and Hikurangi seamounts (HS; white); MHT, mid Havre Trough; SHT, southern Havre Trough. Dashed lines with hexagons are mixing calculations between; (1) depleted mantle wedge and subducted sediments, (2) depleted mantle wedge and Hikurangi Plateau (consisting of 90% average Hikurangi Plateau basement and 10% average Hikurangi seamounts) and (3) subducted sediments and Hikurangi Plateau. See Supplementary Table 1 for modelling details. Hikurangi Plateau and seamount data are from refs 17 , 19 , and this study. Full size image However, if projected beneath the arc, the Rapuhia Scarp subducts approximately beneath the Kibblewhite volcanic centre (~34.2°S; Fig. 1 ). Subduction of an H 2 O-rich, buoyant and thus shallow dipping Hikurangi slab (~20° to ~60 km depth [39] ) is consistent with ~500 m shallowing of the bathymetry, suggesting crustal uplift directly north of Kibblewhite ( cf. ref. 15 ). A more buoyant slab, which hosts bathymetric anomalies (such as LIPs) reducing the overall slab density and thus leading to shallow subduction, has also been predicted by numerical models [40] . The colocated change of the arc lava isotope composition, forearc subsidence, arc front offset into the backarc and deepening seafloor morphology together indicate that the initial Hikurangi Plateau–arc collision could have occurred ~250 km further north near ~32°S (refs 15 , 27 ). Supporting evidence for initial Hikurangi subduction ~250 km further north comes from a satellite-derived Bouguer gravity anomaly of up to ~360 mGal between 32°S and 34.5°S, compared with a regional value of ~240 mGal north and south of the anomaly ( Fig. 4a ), suggesting shallow mantle, or dense mid-lower crust, occurs beneath this region. Two-dimensional gravity modelling along a transect parallel to the Kermadec arc front, from ~30°S to ~35.2°S, indicates maximum crustal thinning at ~32.5°S, gradually thickening both to the north and south from this point. This region of crustal thinning coincides with deeper (by ≤500 m) bathymetry ( Figs 1 and 4b ). The subduction of major ridges or seamounts is one of the most effective mechanisms to increase tectonic erosion [41] . We can therefore assume that the subduction of thickened plateau crust, hosting large seamounts, will significantly increase the rate of tectonic erosion. Much of the margin collapse following removal of plateau support accompanying southward migration of the plateau subduction interface will also enhance effective tectonic erosion [27] . These effects will cause crustal thinning in addition to normal tectonic erosion resulting in the formation of a thick subduction channel mélange at the slab–mantle wedge interface. The apparent increase in crustal thickness towards the south from c. 32.5°, implied by the two-dimensional gravity model ( cf. Fig. 4 ), is likely instead to be partly attributable to dynamic support of the margin (particularly south of 34°) by the subducting buoyant Hikurangi Plateau. Moving southward there is a gradual decrease in the spacing of volcanic edifices along-strike, from one edifice every ~55 km north of ~32°S, to one edifice every ~45 km between ~32° to 35°S and finally to one edifice every ~30 km south of 35°S above the present-day subducting Hikurangi Plateau ( cf. ref. 15 ). This decrease in spacing between volcanic centres is accompanied by an increase in the total volume of lava erupted onto the seafloor from ~830 km 3 between 34°S and 32°S to ~1,200 km 3 between ~35°S and 37°S (ref. 29 ), suggesting not only a relation between Hikurangi Plateau subduction and enhanced magma production, but also an impact on the stress field. That is, enhanced fracturing of the overlying plate, creating relatively more zones of weakness, such as faults in the crust along which magmas are channelled and can rise towards the surface. Dehydration of 15–23-km thick and more H 2 O-rich Hikurangi crust will significantly increase the fluid flux from the subducting plate, thus forming a more hydrated overlying mantle wedge than to the north. 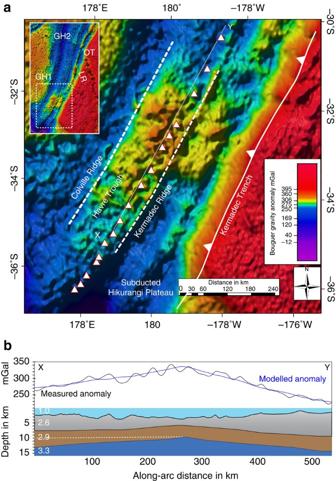Figure 4: Bouguer gravity anomaly map and two-dimensional gravity model along the Kermadec arc front. (a) Satellite-altimetry-derived Bouguer gravity anomaly map of the Kermadec arc system between ~30°S and ~36.5°S. Bouguer gravity anomaly is calculated using free air gravity anomaly (ref.64, version 18) plus NIWA bathymetry65and a 2.67 × 103kg m−3density for the water body. Upper left corner inset shows the Bouguer gravity anomaly for the entire arc. Triangles mark the location of the arc front volcanic centres. White dashed line marks the location of the along-arc profile shown inFig. 4bwith X and Y being the start and end points. GH1, gravity high 1; GH2, gravity high 2 (located where the Louisville seamount chain subducts); LSC, Louisville seamount chain; OT, Osbourn trough. (b) Two-dimensional gravity model along the Kermadec arc front. Dark blue represents the upper mantle overlain by lower crust (brown), upper crust (grey) and seawater (light blue). White numbers are densities in g cm−3. White dashed line within the lower crust marks hypothetical crustal thickness, assuming the addition of dynamic support of the crust from the buoyant Hikurangi Plateau. Figure 4: Bouguer gravity anomaly map and two-dimensional gravity model along the Kermadec arc front. ( a ) Satellite-altimetry-derived Bouguer gravity anomaly map of the Kermadec arc system between ~30°S and ~36.5°S. Bouguer gravity anomaly is calculated using free air gravity anomaly (ref. 64 , version 18) plus NIWA bathymetry [65] and a 2.67 × 10 3 kg m −3 density for the water body. Upper left corner inset shows the Bouguer gravity anomaly for the entire arc. Triangles mark the location of the arc front volcanic centres. White dashed line marks the location of the along-arc profile shown in Fig. 4b with X and Y being the start and end points. GH1, gravity high 1; GH2, gravity high 2 (located where the Louisville seamount chain subducts); LSC, Louisville seamount chain; OT, Osbourn trough. ( b ) Two-dimensional gravity model along the Kermadec arc front. Dark blue represents the upper mantle overlain by lower crust (brown), upper crust (grey) and seawater (light blue). White numbers are densities in g cm −3 . White dashed line within the lower crust marks hypothetical crustal thickness, assuming the addition of dynamic support of the crust from the buoyant Hikurangi Plateau. Full size image Erosion of thickened Hikurangi crust and seamounts and subducted sediments will create a buoyant, H 2 O-rich ‘Hikurangi mélange’, containing a mixture of Hikurangi Plateau basement and seamount material embedded in a metasedimentary matrix including fragments of the overlying crust ( cf. Fig. 5 ). Using a Hikurangi Plateau isotopic composition of 206 Pb/ 204 Pb=19.35; 207 Pb/ 204 Pb=15.62; 208 Pb/ 204 Pb=38.74; 87 Sr/ 86 Sr=0.7037 and 143 Nd/ 144 Nd=0.51295 (see Fig. 3 caption for details), the Pb and Sr isotope signatures in lavas from volcanoes located between ~32 and 35°S can be explained by mixing depleted mantle wedge melts with ~3–10% of subducted sediment and ~20–55% Hikurangi components ( Fig. 3 ). Given that the Kermadec arc is one of the oldest and coldest subduction zones globally with an estimated slab surface temperature of ~745–760 °C beneath ~30.2 to 37.9°S (refs 37 , 42 ), it is unlikely that significant slab melting will occur. Therefore, although Pb and Sr are mobile in aqueous fluids, the decrease in 143 Nd/ 144 Nd values cannot be explained through a subducting slab-derived fluid flux alone (due to low Nd mobility in aqueous fluids at temperatures ≤800° (at 4 GPa; ref. 43 ). Previously, variations in trace element ratios and isotope compositions of rather conservative elements in southern Kermadec arc lavas were attributed to ambient mantle heterogeneity predating the geochemical imprint of the subducting slab [36] . Although ambient mantle wedge heterogeneities (and/or the involvement of deep crustal or lithospheric mantle fragments of rifted Gondwana continental material) could account for the observed isotopic Kermadec arc lava heterogeneities, the simultaneous increase in Pb and Sr but decrease in Nd isotope values, together with the aforementioned observations, plausibly argues for Hikurangi Plateau subduction-related processes causing the observed isotopic changes south of ~32°S. A similar input of an OIB-type slab signature, including a positive gravity anomaly (GH2; Fig. 4a ) can be observed further north, where the subduction of the Louisville Seamount Chain affects the central Tonga–Kermadec arc [14] . 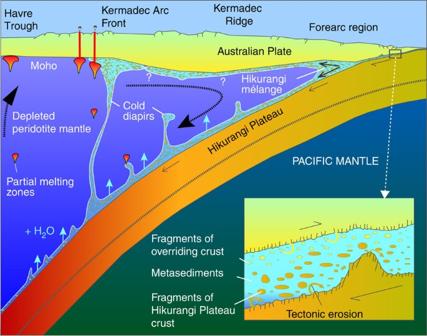Figure 5: Schematic across-arc section. Section illustrating the effect of the subducting Hikurangi Plateau on processes in the mantle and crust beneath the southern Kermadec arc. Increased tectonic erosion in the forearc regions creates a thick, H2O-rich mélange layer, containing fragments of the overriding forearc crust and more importantly of the subducting Hikurangi Plateau in a metasedimentary matrix. The Hikurangi mélange is subducted to deeper depth, where due to its buoyant behaviour forms cold diapirs, which rise through mantle wedge and eventually pond beneath a density barrier, such as the Moho. Because of the dehydration of the subducting plate during its descent, the arc lavas may already contain a fluid-derived (mostly Pb and less significant Sr) Hikurangi Plateau signature. Interaction of melts with the Hikurangi mélange layer at the Moho can also explain the large-scale variation of143Nd/144Nd isotope values not only above the presently subducting Hikurangi Plateau, but also to the north, where the Kermadec arc crust has been underplated in the past. Local variations in lava Sr-, Nd- and Pb-isotope composition may indicate that the Hikurangi mélange does not form a continuous layer beneath the Moho and may only occur locally consistent with its formation through cold diapirs. Figure 5: Schematic across-arc section. Section illustrating the effect of the subducting Hikurangi Plateau on processes in the mantle and crust beneath the southern Kermadec arc. Increased tectonic erosion in the forearc regions creates a thick, H 2 O-rich mélange layer, containing fragments of the overriding forearc crust and more importantly of the subducting Hikurangi Plateau in a metasedimentary matrix. The Hikurangi mélange is subducted to deeper depth, where due to its buoyant behaviour forms cold diapirs, which rise through mantle wedge and eventually pond beneath a density barrier, such as the Moho. Because of the dehydration of the subducting plate during its descent, the arc lavas may already contain a fluid-derived (mostly Pb and less significant Sr) Hikurangi Plateau signature. Interaction of melts with the Hikurangi mélange layer at the Moho can also explain the large-scale variation of 143 Nd/ 144 Nd isotope values not only above the presently subducting Hikurangi Plateau, but also to the north, where the Kermadec arc crust has been underplated in the past. Local variations in lava Sr-, Nd- and Pb-isotope composition may indicate that the Hikurangi mélange does not form a continuous layer beneath the Moho and may only occur locally consistent with its formation through cold diapirs. Full size image Tomography results from a trench-perpendicular ocean bottom seismometer array oriented east-west across the Kermadec trench to the Havre Trough at ~37°S (refs 30 , 31 ) show zones of reduced seismic velocities (that is, Vp ≤7.8 km s −1 compared with ≥8 km s −1 for mantle peridotite) beneath the arc front MOHO, consistent with ≥10% of serpentenized mantle being present beneath the arc [44] . A similar ~10-km thick crust–mantle transition layer with lower seismic velocities (that is, Vp=7.0–7.7 m s −1 ) has also been identified beneath the Izu–Bonin–Mariana and Tonga arcs, interpreted to be composed of a mixture of crustal and mantle materials [45] , [46] . Likewise, beneath the central Taupo Volcanic Zone, a zone of reduced seismic velocities of ≥Vp=7.4 m s −1 (Vp/Vs=~1.87) extends from the Moho to the slab–mantle wedge interface suggesting diapirically rising hydrated and low density material [47] . Lower seismic velocities of Vp=~7.7, (and density=~3.0 g cm −3 ; Vp/Vs=~1.85), which are similar to the velocities observed at the crust–mantle boundary beneath arcs have been measured in exhumed subduction mélange rocks with compositions intermediate between chlorite schists and jadeite (at T=600 °C and P=2 GPa). Numerical modelling results show that buoyant cold diapir formation requires ~1–10-km thick mélange layers at the slab surface–mantle wedge interface (refs 48 , 49 and references therein). The formation of a more hydrated Hikurangi mélange above the subducting plateau than beneath the northern Kermadec arc will reduce the mélange density. This, in turn, is likely to create more diapirs rising through mantle wedge and to partially melt via decompression ( Fig. 5 ). The formation of volatile-rich melts above the subducting Hikurangi Plateau can therefore explain the higher volcano density and possibly the formation of large silicic magma chambers beneath the Taupo Volcanic Zone on the North Island of New Zealand (cf. ref. 50 ). The thin crust between 32 and 34.5°S coincides with the occurrence of large volcanoes, lavas from which show the highest Pb isotopic values, suggesting a high percentage of a Hikurangi component in the mélange formed through increased tectonic erosion during early Hikurangi Plateau subduction. The increasing crustal thickness, 87 Sr/ 86 Sr and 143 Nd/ 144 Nd values but general decrease of 206 Pb/ 204 Pb south of ~35°S indicates the increasing contribution of a sedimentary component gradually diluting the Hikurangi signature. We conclude that a geochemically heterogeneous Hikurangi mélange layer, assimilated by younger ascending, or stagnated Kermadec arc melts, can explain the observed change in arc lava geochemical compositions of the southern Kermadec arc lavas. On the basis of isotopic, bathymetric and gravity variations along the Kermadec arc, the initial arc–Hikurangi Plateau collision can be identified at least 250 km north of its present location, suggesting that a much larger portion of the plateau than previously estimated has been subducted since >10 Myr ( Fig. 6 ). The extent of the gap of the Ontong Java Nui super plateau [22] and of the subducted Hikurangi Plateau portion (inferred by geochemistry, morphology and gravity; Fig. 5 ) suggests that we may have identified the missing piece of this super plateau. Furthermore, we have demonstrated that LIP subduction has profound implications for fundamental processes occurring at oceanic arcs, such as increased rates of tectonic erosion and elevated fluid flux from the subducting slab, which in turn, influence the eruptive behaviour and possibly the style of hydrothermal systems at arc volcanoes and the element transfer into the world’s oceans. 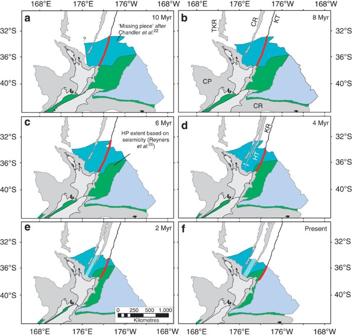Figure 6: GPlates-based reconstruction of Pacific and Australian plates NE of New Zealand. Pacific and Australian Plate (Australian Plate fixed and rigid; Kermadec trench fixed) convergence along the Kermadec arc segment are shown in 2 Myr steps from 10 Myr (a) to present (f) using finite rotations from refs5,66. CP, Challenger Plateau; CR, Chatham Rise; CR, Colville Ridge; HT, Havre Trough; KR, Kermadec Ridge; TKR, Three Kings Ridge. Dark grey areas represent seafloor above ~2,000 m.b.s.l. Red line in each panel indicates the length of Kermadec Trench beneath which Hikurangi Plateau is subducting. Dashed white line marks the Havre Trough. Present extent of the Hikurangi Plateau (light blue shading), present subducted extent derived from seismic tomography and earthquake hypocentres20(green shading), and ‘missing piece’ of Ontong Java Nui (dark blue shading) from ref.22. The reconstruction was conducted using GPlates software available athttp://www.gplates.org/. Figure 6: GPlates-based reconstruction of Pacific and Australian plates NE of New Zealand. Pacific and Australian Plate (Australian Plate fixed and rigid; Kermadec trench fixed) convergence along the Kermadec arc segment are shown in 2 Myr steps from 10 Myr ( a ) to present ( f ) using finite rotations from refs 5 , 66 . CP, Challenger Plateau; CR, Chatham Rise; CR, Colville Ridge; HT, Havre Trough; KR, Kermadec Ridge; TKR, Three Kings Ridge. Dark grey areas represent seafloor above ~2,000 m.b.s.l. Red line in each panel indicates the length of Kermadec Trench beneath which Hikurangi Plateau is subducting. Dashed white line marks the Havre Trough. Present extent of the Hikurangi Plateau (light blue shading), present subducted extent derived from seismic tomography and earthquake hypocentres [20] (green shading), and ‘missing piece’ of Ontong Java Nui (dark blue shading) from ref. 22 . The reconstruction was conducted using GPlates software available at http://www.gplates.org/ . Full size image Sampling The Kermadec arc volcanic centres between ~26°S and 28.6°S (Hinepuia–Hinetapeka) and between ~31°S and 34°S (Havre–Kibblewhite; Fig. 1 ) were mapped and sampled during the RV Tangaroa expeditions NZAPLUME III in 2004 and TAN0205 in 2005 (refs 26 , 33 ). Additional samples from the Hikurangi Plateau (Rapuhia Scarp) were recovered during the R/V Sonne expedition SO168 Zealandia in 2002/2003. Isotope analyses For chemical analysis fresh cores of the samples were extracted, repeatedly washed in deionized water (in an ultrasonic bath) to remove sea salt, then crushed, handpicked and reduced to powder in an agate mill. Isotope analyses were conducted at the University of Melbourne and GEOMAR. At the University of Melbourne between 50 and 100 mg of fresh, clean chips 1–5 mm in diameter were handpicked for isotopic analysis and then leached in hot 6 N HCl for 30 min to remove any contaminants. Samples were then washed in ultrapure water and dissolved in HF/HNO 3 acid mixtures. Separation of Pb, Sr and Nd involved standard ion exchange procedures using Eichron ion specific resins. Analytical blanks are in all cases insignificant relative to the amount of sample processed and no blank corrections were made. Separated Sr, Nd, and Pb were run on a Nu Instruments MC-ICPMS coupled to a CETAC Aridus desolvating nebulizer operating at a sample uptake rate of ~60 μl min −1 . Instrumental mass bias was corrected using an exponential bias law with 87 Sr/ 86 Sr normalized to 86 Sr/ 88 Sr=0.1194 and reported relative to NIST SRM 987=0.710250. For Sr-isotopes, internal precision is typically <0.000015 (2 s.e.) with reproducibility (2 s.d. of repeat runs) ≤±0.000040. 143 Nd/ 144 Nd was normalized to 146 Nd/ 145 Nd=2.0719425 (equivalent to 146 Nd/ 144 Nd=0.7219) and reported relative to La Jolla Nd reference material=0.511865. Internal precision is typically <0.000010 (2 s.e.) with reproducibility (2 s.d. of repeat runs) ≤±0.000020. Pb-isotope ratios are reported relative to SRM 981 values of 16.935, 15.489, 36.701 with reproducibility (2 s.d. of repeat runs) ≤±0.03%. See refs 51 , 52 for Pb and Sr–Nd procedures, respectively. At GEOMAR, leached whole rock powders (6 N HCl at 130 °C for 1 h) were used for Sr, Nd chemistry and leached rock chips (2 N HCl at room temperature for 30 min) for Pb. Sample dissolution involved 4 ml conc. Hf and 1.5 ml HNO 3 at 150 °C for 48 h in a closed teflon vial, followed by evaporation to dryness, uptake in 6 N HCl and final evaporation to dryness. The element chromatography followed established standard procedures [53] . Isotopic ratios were analysed in static multi-collection mode on a TRITON (Nd) and MAT262 RPQ 2+ (Sr–Pb) thermal ionization mass spectrometers. Sr and Nd isotopic ratios are normalized within run to 86 Sr/ 88 Sr=0.1194 and 146 Nd/ 144 Nd=0.7219, respectively and isotope data reported relative to NBS987 87 Sr/ 86 Sr=0.710250±0.000012 (2 s.d., N =20) and 143 Nd/ 144 Nd=0.511850±0.000005 (2 s.d., N =27) for La Jolla. NBS981 gave 206 Pb/ 204 Pb=16.898±0.006, 207 Pb/ 204 Pb=15.437±0.007, 208 Pb/ 204 Pb=36.527±0.024 (2 s.d., N =125; 2003–2006) and were corrected for mass bias to our NBS981 double spike values of 206 Pb/ 204 Pb=16.9412±0.0021, 207 Pb/ 204 Pb=15.4992±0.0020, 208 Pb/ 204 Pb=36.7225±0.0049 (2 s.d., N =69; 2006–2008). This external mass bias procedure applies to samples 34-11 and 36-4 while the remaining samples were mass bias corrected by Pb double spike [54] . Total chemistry were <100 ng Sr–Nd–Pb and thus considered neglible relative to the amount of sample. How to cite this article: Timm, C. et al. Subduction of the oceanic Hikurangi Plateau and its impact on the Kermadec arc. Nat. Commun. 5:4923 doi: 10.1038/ncomms5923 (2014).